Subterranean atmospheres may act as daily methane sinks In recent years, methane (CH 4 ) has received increasing scientific attention because it is the most abundant non-CO 2 atmospheric greenhouse gas (GHG) and controls numerous chemical reactions in the troposphere and stratosphere. However, there is much that is unknown about CH 4 sources and sinks and their evolution over time. Here we show that near-surface cavities in the uppermost vadose zone are now actively removing atmospheric CH 4 . Through seasonal geochemical tracing of air in the atmosphere, soil and underground at diverse geographic and climatic locations in Spain, our results show that complete consumption of CH 4 is favoured in the subsurface atmosphere under near vapour-saturation conditions and without significant intervention of methanotrophic bacteria. Overall, our results indicate that subterranean atmospheres may be acting as sinks for atmospheric CH 4 on a daily scale. However, this terrestrial sink has not yet been considered in CH 4 budget balances. Methane (CH 4 ) is currently the most abundant non-CO 2 greenhouse gas (GHG) in the atmosphere, reaching a global average concentration of ∼ 1,800 p.p.b. at mid-northern latitudes [1] . Despite significant research progress in recent years, large uncertainties remain about the CH 4 budget and its evolution over time because there is a lack of knowledge about CH 4 sinks and sources [2] , [3] , [4] , [5] . Superimposed on the long-term trend of increasing atmospheric CH 4 , there is significant interannual variability [1] , [6] , [7] , and the sources of variation remain controversial [8] . Current CH 4 estimates account for ∼ 22% of the total forcing potential of all long-lived GHGs [9] . By weight, CH 4 is 28 times more effective at trapping heat in the atmosphere than CO 2 over a 100-year period [10] . Sensible mitigation strategies also require a quantitative understanding of the CH 4 budget regarding emissions and sinks [11] . The total global emissions of CH 4 are constrained reasonably well by atmospheric observations and estimates of its lifetime, based on multiple atmospheric CH 4 inversion models (top–down studies). However, the uncertainties concerning emissions/consumption from individual sources/sinks [12] are greater, and they are poorly constrained by the current atmospheric observation network [6] . Some unaccounted sinks (or sources) could contribute the global CH 4 budget and its long-term variations. The Earth’s surface exerts its influence on the free atmosphere through the atmospheric boundary layer. This lowest portion of the atmosphere ranges from a few tens of metres to 1–2-km deep [13] . The subsurface atmosphere is usually overlooked as an important part of this boundary layer. At the top of the subsurface layer in the vadose zone (below the subsoil and above the groundwater table) highly specific biogeochemical processes occur, which may act as regulators of gas exchanges between the surface and the free atmosphere. The uppermost part of the vadose zone may contain large amounts of underground air, that is, a CO 2 -rich air reservoir permeating the unsaturated zone [14] . Underground air occupies air-filled caves, empty-water pores, cracks and voids in bedrock or unconsolidated sediment, some of which exhibit a direct connection to the open atmosphere [15] . The gas exchange between the bulk of the atmosphere and small air-filled locations, for example, fissures, cracks and voids, is minor compared with the exchange that occurs between large shallow caves and the open atmosphere. Hence, shallow caves can be thought of as small-scale representations of the uppermost part of the vadose zone, where there is intense gas exchange with the atmosphere. Shallow caves may largely represent the volume of underground air that is distributed widely across continental ecosystems. Furthermore, shallow caves are favourable for in situ monitoring of gaseous exchange processes at the subsurface. They are easily accessible natural macropores that can store edaphic or atmospheric gases several tens of metres below the soil. These shallow vadose environments below the soil show significant seasonal and even daily variations in the gas composition of underground air [16] , [17] , [18] , which involves the exchange of large amounts of other GHGs in addition to CO 2 (g) with the lower troposphere [15] , [19] . However, there is great uncertainty regarding the behaviour and lifetime of CH 4 in these shallow vadose environments. Here to better understand the behaviour and lifetime of the CH 4 in subsurface environments located in the vadose zone, spatiotemporal spot measurements and continuous geochemical tracing of air (in the atmosphere, soil and cave air) have been carried out by monitoring CH 4 , CO 2 and stable carbon isotopic δ 13 C[CO 2 ] using cavity ring-down spectroscopy (CRDS). In total, >1,000 air samples have been analysed for seven caves located in Spain. 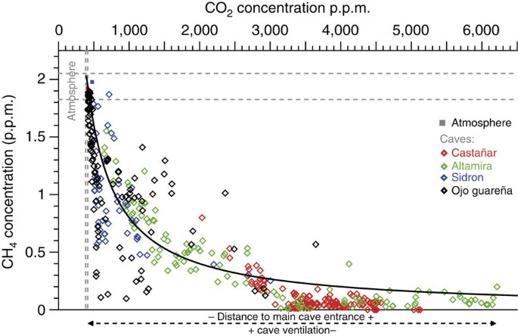Figure 1: Variations in the concentrations of GHGs in underground air. Caves (open diamonds), local atmosphere (solid squares). The grey dashed lines indicate the regional levels of the atmospheric CH4and CO2Dry Air Mole Fractions from the NOAA earth system research laboratory (ESRL) global monitoring division (GMD) Carbon Cycle Cooperative Global Air Sampling Network as a reference62,63. In particular, the grey dashed lines correspond to representative minimum and maximum data from the well-mixed troposphere from central Spain (Centro de Investigación de la Baja Atmósfera, University of Valladolid, 41.81° N, 4.93° W, 845 m a.s.l. (above sea level)) for the period 2011–2012 coeval to the cave air samplings. The caves exhibit a wide range of geographic, geologic and climatic features ( Supplementary Table 1 ). For each cave, the sampling was conducted in underground air, soil air and external atmosphere. Comprehensive microclimatic monitoring of the exterior, soil and cave atmosphere was conducted simultaneously with GHG tracking. In addition, potential methanotrophy at each subsurface site was assessed by tracking the presence of methane-oxidizing bacteria (MOB) using specific DNA primers for methanotroph pmoA sequences [20] . The overall results show that complete consumption of CH 4 is favoured in the subsurface atmosphere under near vapour-saturation conditions without significant intervention of methanotrophic bacteria. The oxidative capacity of underground air must be related to its high density of ions, some of which are likely to react with CH 4 . Overall, our results indicate that subterranean atmospheres may be acting as sinks for atmospheric CH 4 on seasonal and daily scales. GHGs in underground air Spot air samplings were conducted during short surveys at all fieldwork sites, within a predefined network of points that were spatially distributed from the entrance to the innermost accessible areas of the cavities. Exterior and soil air were also sampled at fixed locations throughout the day, and, preferably, during maximum (midday) and minimum photosynthetic activity (early morning). Further details about the air-sampling procedures are found in Methods section. Air samples were analysed in the laboratory within 48 h of sampling for determine CO 2 and CH 4 concentrations and the isotopic δ 13 CO 2 signal using CRDS technology. The comparison of CO 2 and CH 4 enables assessment of the influence of the exterior atmosphere and soil on the gas contents of cave air, that is, the degree of isolation of the subsurface environment. Figure 1 shows the variations in the concentration of CH 4 and CO 2 in underground air relative to their local atmospheric levels for the main four caves studied. Supplementary Figure 1 shows the extended results for the entire set of caves studied, covering a wide latitudinal transect of the Iberian Peninsula that includes different environmental features, which are summarized in Supplementary Table 1 . There is an inverse relationship between the two GHGs along a subsurface–soil–atmosphere profile. Both soil and cave air exhibit a lower concentration of CH 4 compared with local atmospheric background and regional CH 4 levels (1.83–2.05 p.p.m. for the period 2011–2012, based on records for Central Spain from NOAA). An opposite pattern is found for CO 2 in cave air, which is consistent with the usual magnitude of the CO 2 (g) reservoirs found in shallow caves [21] , [22] , presenting average values that are 10–100 times the current mean atmospheric concentration (0.04% vol). The overall results indicate a higher CH 4 depletion rate (from −0.1 to −0.4 p.p.m. for each 100 p.p.m. increase in CO 2 ) under low-moderate contents of CO 2 (<1,000 p.p.m.). Furthermore, this CH 4 depletion rate rises in highly ventilated caves (for example, the Ojo Guareña and Sidron caves) within a narrow increment of CO 2 (500→700 p.p.m.). Shallow caves where there is intermediate and seasonal ventilation of underground air (for example, the Altamira Cave) display a lower rate of decreases in CH 4 contents (lower than −0.1 p.p.m. of CH 4 for each 100 p.p.m. increment of CO 2 ), especially in cave locations subjected to a stronger influence of the external atmosphere, but showing considerable CO 2 levels (1,000–3,000 p.p.m.). Most isolated caves with the lowest ventilation rates (for example, the Castañar Cave) present a steady state, with practically null CH 4 levels, thus suggesting that complete removal of CH 4 from the underground air occurs once a CO 2 concentration above 3,000 p.p.m. is reached, which is observable in the deepest remote cave locations. The dynamically ventilated caves show greater spatiotemporal variability in their CO 2 and CH 4 concentrations, which is shown by the fact that the paired data for both the parameters are more scattered compared with caves in which there is limited ventilation of underground air. Figure 1: Variations in the concentrations of GHGs in underground air. Caves (open diamonds), local atmosphere (solid squares). The grey dashed lines indicate the regional levels of the atmospheric CH 4 and CO 2 Dry Air Mole Fractions from the NOAA earth system research laboratory (ESRL) global monitoring division (GMD) Carbon Cycle Cooperative Global Air Sampling Network as a reference [62] , [63] . In particular, the grey dashed lines correspond to representative minimum and maximum data from the well-mixed troposphere from central Spain (Centro de Investigación de la Baja Atmósfera, University of Valladolid, 41.81° N, 4.93° W, 845 m a.s.l. (above sea level)) for the period 2011–2012 coeval to the cave air samplings. Full size image The CH 4 depletion rate and its variation relative to CO 2 content in underground air ( Fig. 1 ) were, therefore, key parameters for assessing the ventilation of subterranean atmospheres. In highly ventilated caves, a significant volume of air circulates daily, and, consequently, there is a nearly continual contribution of air to the subterranean atmosphere, which has lower CO 2 content and atmospheric levels of CH 4 . Hence, the CH 4 depletion rises with slight changes in CO 2 close to atmospheric background. Conversely, in the most isolated caves, CO 2 reaches high concentrations because air exchange with the outer atmosphere is negligible. Thus, the removed CH 4 is not rapidly replenished. As a result, the CH 4 depletion rate tends to become negligible as the CO 2 content of cave air rises. The CO 2 concentration in cave air is determined by the mixing of background atmospheric CO 2 with soil-produced CO 2 , and the mixing process fits a Keeling model with a mean y -intercept value ranging from −25 to −28‰ for the caves studied ( Fig. 2 ). The CO 2 -soil recharge by diffusion is more of an important factor at the most isolated subterranean sites, such as Castañar and Altamira caves, where the cave air usually has a higher CO 2 concentration and δ 13 C[CO 2 ] below −20‰ with respect to other caves. Conversely, the lower CO 2 concentration and the δ 13 C[CO 2 ] value that tends toward the local atmospheric background ( ∼ 9%), as measured in Sidron and Ojo Guareña caves, indicates rapid air renewal that allows the air to become well-mixed with the atmosphere. 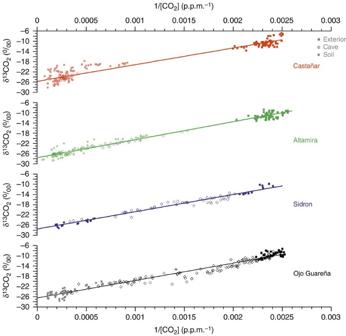Figure 2: Keeling models for the subterranean atmosphere at each cave site. Isotope ratios are plotted against the inverse of CO2concentration for all air samples (seeSupplementary Table 1, and notice the number of air samples for each fieldwork site), distinguishing a three-component mixture: background atmosphere (solid squares), cave air (open diamonds) and soil air (solid circles). The y-intercept of the Keeling models corresponds to the carbon isotope composition for the integrated value of the CO2sources in the ecosystem: −25.71‰ for Castañar cave (R2=0.93), −27.59‰ for Altamira cave (R2=0.98), −27.50‰ for Sidron cave (R2=0.97) and −26.48‰ for Ojo Guareña cave (R2=0.96). As the distance of the cave air samples from the y-intercept of the Keeling models increases, there is greater ventilation and greater influence of the external atmosphere. Conversely, when CO2concentration is high and δ13C[CO2] tends toward the y-intercept, the gas enters by diffusion and has a mainly edaphic origin. Figure 2: Keeling models for the subterranean atmosphere at each cave site. Isotope ratios are plotted against the inverse of CO 2 concentration for all air samples (see Supplementary Table 1 , and notice the number of air samples for each fieldwork site), distinguishing a three-component mixture: background atmosphere (solid squares), cave air (open diamonds) and soil air (solid circles). The y-intercept of the Keeling models corresponds to the carbon isotope composition for the integrated value of the CO 2 sources in the ecosystem: −25.71‰ for Castañar cave ( R 2 =0.93), −27.59‰ for Altamira cave ( R 2 =0.98), −27.50‰ for Sidron cave ( R 2 =0.97) and −26.48‰ for Ojo Guareña cave ( R 2 =0.96). As the distance of the cave air samples from the y-intercept of the Keeling models increases, there is greater ventilation and greater influence of the external atmosphere. Conversely, when CO 2 concentration is high and δ 13 C[CO 2 ] tends toward the y-intercept, the gas enters by diffusion and has a mainly edaphic origin. Full size image Seasonal variation of CH 4 in dynamically ventilated caves Multi-parameter monitoring was conducted for the cave–soil–atmosphere (main climatic data and gas composition) and geochemical tracing was performed using δ 13 C–CO 2 to assess the climate-driven fluctuations of GHGs in the subsurface and to determine the spatiotemporal patterns of exchange between soil and atmosphere. A 3-km-long area of the subterranean system of Ojo Guareña (northern Spain) was chosen for field research. The Ojo Guareña cave system is one of the longest caves in Europe and is the most dynamically ventilated cave site of all the sites studied, according to our most recent studies [23] . Cave air ventilation increased from the end of the summer to early winter in the case of the Ojo Guareña subterranean system ( Fig. 3 ; Supplementary Fig. 2 ). During winter, the outside air temperature is lower than the inside air temperature, and, consequently, the outside air density is higher than the cave air density. This favours advective air movement, primarily through the cave entrance and other host-rock discontinuities. Therefore, a higher proportion of CH 4 -enriched air was progressively transferred from the open atmosphere to the cave during the winter months than in summer. Higher CH 4 depletion with narrow increases of CO 2 indicates a prevailing influx of outer air into the cave, and the CH 4 consumption rate consequently increases from summer to winter. The CH 4 depletion rate in underground air with an increasing CO 2 concentration is significantly higher than the rate of CH 4 consumption through soil MOB. The CH 4 depletion, coeval to increments of CO 2 concentration in underground air, is higher in cave locations that are closer to the surface (CH 4 concentration above 0.75 p.p.m.) and decreases in deeper and more isolated locations (CH 4 concentration below 0.5 p.p.m.). In the most isolated locations, CO 2 diffusion from the soil prevails over the influx of exterior air with the atmospheric CH 4 levels and lower CO 2 concentrations. 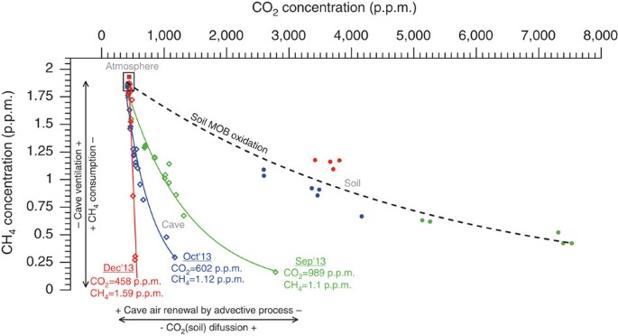Figure 3: Seasonal variability of GHGs in a dynamically ventilated cave. Cave (Ojo Guareña, Spain) air samples (open diamonds), soil air samples (solid circles) and atmospheric air samples (solid squares). Each colour corresponds to an air sampling date in 2013: September (green), October (blue) and December (red). The dashed black line represents CH4oxidation by soil MOBs as a function of CO2concentration in the soil air ([CH4, p.p.m.]=2.04 × exp(−2.09 × 10−4× [CO2, p.p.m.]),R2=0.96). Coloured lines correspond to the functions for each monthly set of paired CH4and CO2data for the air from cave environments; 18 September 2013: [CH4, p.p.m.]=2.72 × exp(−9.95 × 10−4× [CO2, p.p.m.]),R2=0.98), 29 October 2013: [CH4, p.p.m.]=4.35 × exp(−2.3 × 10−3× [CO2, p.p.m.]),R2=0.96) and 10 December 2013: [CH4, p.p.m.]=−1.35 × 10−2× [CO2, p.p.m.]+7.79,R2=0.82. The slope of these coloured lines is indicative of the consumption of atmospheric CH4due to the influx of outer air into the cave via advective processes. In the case of the exponential functions, an increase of the coefficient multiplying the CO2concentration implies a higher CH4depletion. The average concentrations of CH4and CO2in underground air for each month is indicated, considering the entire set of 15 cave-air-sampling points for each field campaign. Figure 3: Seasonal variability of GHGs in a dynamically ventilated cave. Cave (Ojo Guareña, Spain) air samples (open diamonds), soil air samples (solid circles) and atmospheric air samples (solid squares). Each colour corresponds to an air sampling date in 2013: September (green), October (blue) and December (red). The dashed black line represents CH 4 oxidation by soil MOBs as a function of CO 2 concentration in the soil air ([CH 4 , p.p.m. ]=2.04 × exp(−2.09 × 10 −4 × [CO 2 , p.p.m. ]), R 2 =0.96). Coloured lines correspond to the functions for each monthly set of paired CH 4 and CO 2 data for the air from cave environments; 18 September 2013: [CH 4 , p.p.m. ]=2.72 × exp(−9.95 × 10 −4 × [CO 2 , p.p.m. ]), R 2 =0.98), 29 October 2013: [CH 4 , p.p.m. ]=4.35 × exp(−2.3 × 10 −3 × [CO 2 , p.p.m. ]), R 2 =0.96) and 10 December 2013: [CH 4 , p.p.m. ]=−1.35 × 10 −2 × [CO 2 , p.p.m. ]+7.79, R 2 =0.82. The slope of these coloured lines is indicative of the consumption of atmospheric CH 4 due to the influx of outer air into the cave via advective processes. In the case of the exponential functions, an increase of the coefficient multiplying the CO 2 concentration implies a higher CH 4 depletion. The average concentrations of CH 4 and CO 2 in underground air for each month is indicated, considering the entire set of 15 cave-air-sampling points for each field campaign. Full size image Daily variation of CH 4 consumption in ventilated caves In situ and real-time measurements of CO 2 , CH 4 and δ 13 CO 2 were carried out during an intensive field campaign in Altamira Cave. This intensive monitoring period was examined to assess the complete daily cycles of the GHG mixing ratios through comprehensive real-time logging using the same field-deployable CRDS analyser. The results summarized in Fig. 4 correspond to data records from the field campaign conducted in September 2011 (end of summer). In Methods section are summarized the technical procedures applied in the real-time air monitoring deployed in the field sites, including the number and frequency of records and the δ 13 C–CO 2 calculation. 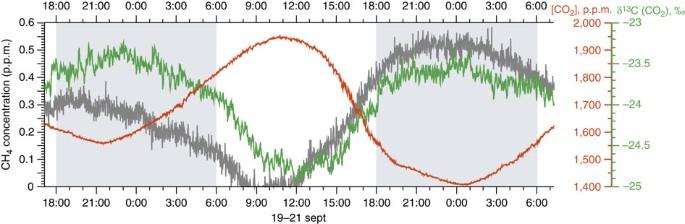Figure 4: Daily variations of CH4and CO2contents and the carbon isotopic signal in underground air. Data from the Altamira Cave (from day 19 to 21 September 2011). The shaded area represents the night-time period delimited by null solar radiation, in accordance with ancillary monitoring parameters (the applied methods and full time series are described by Garcia-Antonet al.18). All records are reported relative to Greenwich Mean Time. Figure 4: Daily variations of CH 4 and CO 2 contents and the carbon isotopic signal in underground air. Data from the Altamira Cave (from day 19 to 21 September 2011). The shaded area represents the night-time period delimited by null solar radiation, in accordance with ancillary monitoring parameters (the applied methods and full time series are described by Garcia-Anton et al. [18] ). All records are reported relative to Greenwich Mean Time. Full size image The interaction of three air masses (soil–cave–exterior) is driven by soil-derived CO 2 diffusion into the cave and by the advective mixing of the cave with exterior air [18] . The diffusive process increases cave CO 2 concentration and decreases δ 13 C[CO 2 ], to the extent that biological respiration in the soil causes an accumulation of CO 2 molecules with a lighter carbon isotopic signature. In contrast, advective mixing causes the CO 2 levels to decrease and causes the isotopic signal to increase because it causes the uptake of air with an atmospheric CO 2 level and a heavier δ 13 C[CO 2 ] compared with both soil and cave air. The diffusive flux usually increases with soil CO 2 production, and the advective flux is driven by outer–inner density gradients. Both of these drivers are primarily regulated by the external meteorological conditions. The monitoring results confirmed that the driving forces for the increases in CH 4 in underground air are the same as for the declines in CO 2 levels, and the daytime increase of the CH 4 content of underground air (+0.04 p.p.m. h −1 on average with the maximum reaching +0.11 p.p.m. h −1 ) is, therefore, synchronous with decline in the CO 2 levels and an increase in δ 13 C[CO2] ( Fig. 4 ), which points to an air inlet from the outside atmosphere. Consequently, the maximum values of CH 4 begin to be reached after sunset but usually remain below the background atmospheric levels. On the contrary, during the night, the CH 4 depletion of underground air is coeval with an increase in CO 2 contents and a decrease in δ 13 C[CO2], which indicates the existence of a CO 2 gas inlet with an edaphic origin, primarily via diffusion. Conversely, the gradient of CH 4 contents between the soil and cave is not sufficient to enable an influx to underground air, due to the likely CH 4 consumption in soil through MOBs action. In the absence of nocturnal influx of atmospheric CH 4 via advective forces, CH 4 consumption mechanisms in the underground air seem to be triggered, the CH 4 content consequently decreases to an average rate of −0.03 p.p.m. h −1 (maximum of −0.05 p.p.m. h −1 ), reaching 0 p.p.m. early in the morning (8:30 h Greenwich Mean Time). Tracking the presence of MOB We evaluated whether the CH 4 oxidation pattern by soil MOB was repeated in cave sediments. Microbiological sampling was conducted to assess the presence or absence of MOBs in the edaphic profile at the exterior and in sediments and on rock surfaces in the cave at each monitored field site. The collected samples were analysed through an ordered set of techniques, including nucleic acid extraction and PCR amplification, cloning and sequencing and sequence analyses (see Methods section for details of these analytical techniques). The results obtained through microbiological sampling of cave sediments from the main four caves studied revealed the presence of Methylocapsa aurea (FN433470), Methylomicrobium album (EU722431) , Methylococcus capsulatus (AE017282) and methanotrophs of the K1-1 (AF547174) and K3-16 (AF547178) strains only in the samples from the Altamira, Sidron and Ojo Guareña caves, mainly in locations where CH 4 usually reaches concentrations near to the atmospheric background levels. These analyses did not detect methanotrophs in remote subterranean locations or poorly ventilated caves, such as the Castañar Cave, where CH 4 is absent or present in minimal concentrations (below the accuracy threshold) throughout the year. CH 4 removal in relation to other environmental parameters Our initial measurements of the density of ions in Castañar Cave (roughly 200 × 10 3 ions per cm 3 ) revealed an extraordinary degree of air ionisation, ∼ 100–1,000 times greater than in the local open atmosphere. The high density of ions in this cave atmosphere persists throughout the year, in the absence of CH 4 . This leads us to hypothesize that the oxidative capacity of underground air is related to its high density of ions, some of which likely are able to react with CH 4 . In light of these preliminary observations, a specific and detailed multiparametric field study was conducted in the cave that had the highest ventilation rate, Ojo Guareña Cave [23] . This underground system was chosen because positive concentrations of CH 4 were always recorded throughout the year, in contrast to other isolated underground sites such as Castañar Cave. In Castañar Cave, CH 4 is hardly detected at all throughout the annual cycle. The field study included the monitoring of gas composition (air ion concentration, CH 4 , CO 2 and its carbon isotopic signal) and microclimatic parameters (temperature and relative humidity). Spot air sampling was conducted during a short survey of the cave air, soil air and open atmosphere using the same procedures described above. The density of ions in underground air as measured simultaneously with environmental monitoring and air sampling using a handled air ion counter (AlphaLab Air Ion Counter, UT, USA). 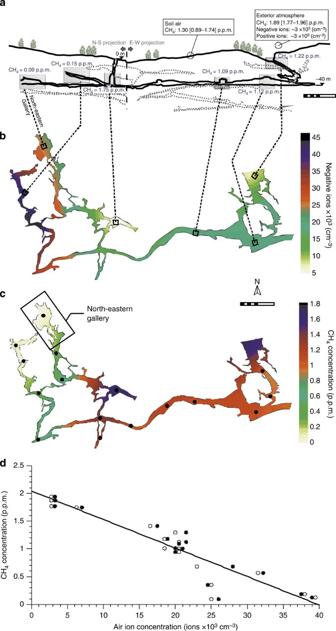Figure 5: Spatial variation of air ion concentration and CH4concentration in underground air. Data from a dynamically ventilated cave (Ojo Guareña, Spain). Sampling campaign of 8 October 2014. Length of scale bars is 50 m. (a) Detailed cross-sections of cave galleries in relation to surface geomorphology and the main entrances to the subterranean system (solid black line represents the studied galleries; the ends of these galleries continue with the rest of the subterranean system, which is not drawn; and the dotted lines show the locations of other cave levels). Data on air ion and CH4concentrations in the atmosphere and in soil air are displayed in relation to the average CH4concentration of the main cave sectors (shaded rectangles). (b) Spatial distribution of negative ions (both negative and positive ions have the same range of concentration, 5–45 × 103ions per cm3, and an identical spatial distribution. Thus, only the spatial distribution of the negative ions is displayed to avoid redundancy). (c) Spatial distribution of CH4, indicating a network of points (filled black circles) at which spot sampling of cave air was conducted. CH4data come from the spot air sampling during short surveys and the subsequently GHG analyses on lab using the CRDS technique. The spatial maps for each parameter were constructed using geostatistical gridding based on an ordinary point kriging method, with a linear variogram model and without anisotropy constraints during interpolation (distance between the estimated points ranging from 3 to 5 m). The north-eastern gallery connected with the rest of the subterranean system is shown in both maps. (d) Functional relationship between air ion concentration (open circles: negative ions and closed circles: positive ions) and CH4concentration in underground air. The continuous black line corresponds to a linear function that best fits the prevailing CH4depletion in the underground air, which occurs as the air becomes increasingly ionized ([CH4, p.p.m.]=−0.051 × [ions × 103, cm−3]+2.04, withR2=0.87). Air ion concentration refers to either positive ions or negative ions. Figure 5 summarizes the spatial variation of air ion concentration and CH 4 content in the underground air of Ojo Guareña Cave. The negative and positive ions have the same concentration range (5–45 × 10 3 ions per cm 3 ) and an identical spatial distribution. Hence, Fig. 5 includes only the spatial distribution of negative ions (the positive ions show the same distribution). The spatial distributions of other ancillary parameters are displayed in Supplementary Fig. 3 , including air temperature, CO 2 concentration and CO 2 carbon isotopic signal, δ 13 C[CO 2 ] (the relative humidity of cave air remains close to a steady state of saturation, 100%, in the entire network of air-sampling points). Radon concentration in the air was continuously monitored in two cave locations with opposite ventilation patterns [23] . The levels of radon observed during the 24-h cycle immediately before the fieldwork campaign ranged from 693 [454–1,033] Bq m −3 , at the final stretch of the western gallery near the cave entrance, to 966 [760–1,386] Bq m −3 in the dead-end gallery located in the northeast sector of the subterranean system ( Fig. 5a ). Figure 5: Spatial variation of air ion concentration and CH 4 concentration in underground air. Data from a dynamically ventilated cave (Ojo Guareña, Spain). Sampling campaign of 8 October 2014. Length of scale bars is 50 m. ( a ) Detailed cross-sections of cave galleries in relation to surface geomorphology and the main entrances to the subterranean system (solid black line represents the studied galleries; the ends of these galleries continue with the rest of the subterranean system, which is not drawn; and the dotted lines show the locations of other cave levels). Data on air ion and CH 4 concentrations in the atmosphere and in soil air are displayed in relation to the average CH 4 concentration of the main cave sectors (shaded rectangles). ( b ) Spatial distribution of negative ions (both negative and positive ions have the same range of concentration, 5–45 × 10 3 ions per cm 3 , and an identical spatial distribution. Thus, only the spatial distribution of the negative ions is displayed to avoid redundancy). ( c ) Spatial distribution of CH 4 , indicating a network of points (filled black circles) at which spot sampling of cave air was conducted. CH 4 data come from the spot air sampling during short surveys and the subsequently GHG analyses on lab using the CRDS technique. The spatial maps for each parameter were constructed using geostatistical gridding based on an ordinary point kriging method, with a linear variogram model and without anisotropy constraints during interpolation (distance between the estimated points ranging from 3 to 5 m). The north-eastern gallery connected with the rest of the subterranean system is shown in both maps. ( d ) Functional relationship between air ion concentration (open circles: negative ions and closed circles: positive ions) and CH 4 concentration in underground air. The continuous black line corresponds to a linear function that best fits the prevailing CH 4 depletion in the underground air, which occurs as the air becomes increasingly ionized ([CH 4 , p.p.m. ]=−0.051 × [ions × 10 3 , cm −3 ]+2.04, with R 2 =0.87). Air ion concentration refers to either positive ions or negative ions. Full size image The minimum air ion concentrations, for both negative and positive ions, were measured close to the cave entrances, with values slightly higher than those observed in the exterior atmosphere. Medium values (15–25 × 10 3 ions per cm 3 ) were measured in the cave sector between the entrances, where bidirectional air circulation is noticeable throughout the year, accordingly to our continuous monitoring studies [23] . The highest ionisation levels of cave air were found in the eastern dead-end gallery of the cave, coinciding with the highest CO 2 (>2,500 p.p.m.) concentration, the lowest levels of δ 13 C[CO 2 ] (<−23‰) ( Supplementary Fig. 3 ) and the maximum radon activity in the air, which indicates less influence of the aerodynamic processes that control cave air renewal. The spatial pattern of CH 4 concentration is the opposite of the air ion concentration pattern ( Fig. 5d ). In accordance with the estimated spatial distribution of the CH 4 content in underground air, ∼ 80% of the cave surface ( ∼ 7,160 m 2 ) has a CH 4 concentration below the levels found in soil air (0.89–1.74 p.p.m. ), with almost null values in the north-eastern galleries far from the cave entrances. The remaining 20% of the cave surface is located near entrances and has the CH 4 levels close to the local atmospheric background (1.77–1.96 p.p.m.). The atmospheric CH 4 is reduced to ∼ 1 p.p.m. when moving from the accesses to the subterranean system to the highly ventilated sector between both cave entrances. A linear function fits the data describing CH 4 depletion in the underground air as it becomes increasingly ionized ( Fig. 5d ). A CH 4 removal of 0.26 p.p.m. in the subsurface atmosphere is observed as the air ion concentrations, both positive and negative, increase to 5 × 10 3 ions per cm 3 . Depletion of local atmospheric CH 4 ranging from 1.17 to 1.36 p.p.m. is expected based on the averaged degree of ionisation of the subsurface atmosphere at the fieldwork site ( ∼ 23.3 ions·per cm 3 , for both positive and negative ions). Some points differ to this linear trend, that is, they show a low CH 4 concentration, below 1 p.p.m., with an intermediate air ion concentration ( ∼ 25 × 10 3 ions·per cm 3 ; Fig. 5d ). These points correspond to air-sampling points located in a north-eastern gallery connected with the rest of the subterranean system ( Fig. 5 ). This cave sector is under the influence of air exchange processes that cause an influx of underground air that is heavily depleted in CH 4 , but less ionized than the bordering galleries with similar minimum CH 4 concentrations. Therefore, this intermediate air ion concentration ( ∼ 25 × 10 3 ions·per cm 3 ) seems to be enough to cause CH 4 concentrations below 0.5 p.p.m. The values of the ancillary key parameters (lower air temperature, higher CO 2 content and a reduced δ 13 C[CO 2 ] signal, as shown in Supplementary Fig. 3 ) confirm the distinctive higher ventilation of this cave sector relative to the surrounding galleries. The northernmost galleries with no air circulation are less influenced by the air renewal processes and that affects their maximum air ion concentration and minimum CH 4 concentration. The CH 4 consumption in underground air is markedly higher than CH 4 depletion in soil air due to methanotrophy. In addition, the CH 4 consumption rate in underground air varies depending on the CH 4 input ratio from the atmosphere, which is determined by the intensity of cave air ventilation represented by the CO 2 levels. Real-time measurements have revealed that consumption of atmospheric CH 4 in subsurface environments is even faster than at the soil surface, within just a few hours. Thus, the CH 4 concentration in underground air varies throughout day, showing a very similar pattern to the carbon isotope δ 13 C[CO 2 ] signal, but presenting an opposite pattern to CO 2 contents. In the case of CO 2 , its movement occurs through a combination of advection and diffusion processes, at both daily [17] , [18] and seasonal [24] , [25] timescale. The outer air that enters the cave, mainly during daylight hours, is fully depleted of CH 4 within a few hours, and this underground air reservoir subsequently partially advects upwards and exhales out into the atmosphere on a daily basis. Therefore, the variation in CH 4 abundance reveals itself as a key parameter for assessing the ventilation of subterranean atmospheres, as in the case of other tracer gases (radon). This circadian pattern of both GHGs has been consistently observed over different seasons, and, preferentially, in dynamically ventilated caves during periods of the year with drier conditions. These results are fully consistent with the subsurface environments acting, at a short-term scale, as cleaning filter for atmospheric CH 4 coming from air that directly enters the subsurface, bypassing the edaphic layer via air mass advection (for example, through a cave entrance), far from the influence of biochemical oxidation by soil CH 4 and methanotrophic bacteria. The main mechanism responsible for the complete consumption of CH 4 in the studied underground environments must be something other than the previously suggested bacterial oxidation mechanism [26] , [27] because the remaining null CH 4 concentration is not sufficient to satisfy energy requirements for the maintenance and growth of methanotrophic populations. In our MOB tracking, we did not detect methanotrophs in the cave sediments from poorly ventilated subterranean sites. This is consistent with the fact that we found no significant concentrations of CH 4 throughout the year. This suggests that an agent other than methanotrophs should also consume CH 4 at subsurface locations where the gas is absent for long periods. A negative correlation between CH 4 concentration and the density of ions in the cave air has been observed in highly ventilated caves (for example, Ojo Guareña). In this context, charged airborne particles with electrical mobility (primarily, inorganic ions) could play a significant oxidizing role. The small ions exist all the time in the atmosphere, and the average concentrations of positive and negative small ions are typically 0.2–2.5 × 10 3 cm −3 (ref. 28 ). However, concentrations up to 45 × 10 3 cm −3 have been observed in the dynamically ventilated caves studied (for example, the Ojo Guareña Cave). Some anomalous high concentrations of ions have previously been reported in other underground locations [29] . During their lifetime of about 100 s, small ions undergo a series of ion-molecule reactions and continuously change their chemical identity [30] . The negative ions have greater affinity for the condensing vapours [31] , [32] , consequently the ion-mediated particle formation mechanisms are expected to be important in locations with high relative humidity [33] , [34] , close to 100% (for example, in caves). The small air ions are usually composed of the central primary ion and surrounding 4–10 molecules of water, depending on humidity, temperature, actual concentration of trace gasses [35] and polarity of the ions. The main natural sources of small ions are air molecule ionization by radon decay, gamma and cosmic radiation, all of them exhibiting strong spatial and temporal variations [28] . The enhanced radon activity concentration causes the variation in the ionization rate, increasing the small ion concentrations observed near the ground at certain sites, especially where there is an accumulation of radon in the air [29] , [36] , [37] , [38] . The ionization rate via radon decay is highly sensitive to the elevation from the ground, so it is larger closer to the ground [39] . Recent indoor experiments showed that determining positive air ion concentration could be an alternative method for evaluating radon activity concentrations [40] . It has been also observed that the source rate of small ions by radon activity is elevated indoors ( ∼ 12 ion pairs per cm 3 s −1 ), with concentrations that follow diurnal cycles affected by ventilation. The highest concentrations are observed at night, when there is little or no ventilation [30] , [41] . In this regard, caves are suitable locations to storing underground air with high radon activity [42] , particularly, when the underground atmosphere has a low air renewal rate (for example, Castañar Cave [16] , [43] ). It is expected that there will be a high density of ions in such environments, and this is borne out by the measurements made in the subterranean sites that were studied. The results derived from our continuous monitoring of radon activity in underground air confirm that CH 4 depletion occurs in underground air as it is enriched in radon ( Fig. 6 ). The ratio of the concentrations of CO 2 and CH 4 is directly proportional to the intensity of ventilation process of the subsurface atmosphere, that is, the degree of cave air renewal through the inlet of air from exterior with the atmospheric levels of both the gases (CO 2 and CH 4 ). The ratio of the concentrations of CO 2 and CH 4 tends to zero once the radon concentration in underground air exceeds 2,000 Bq m −3 ( Fig. 6 ). 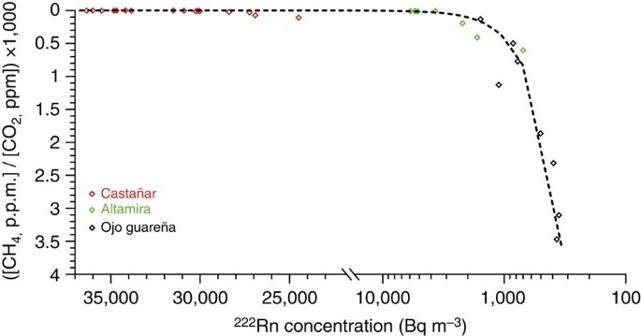Figure 6: Variation in the ratio of the concentrations of both greenhouse gases in underground air in relation to radon activity. The ratio of the concentrations of CO2and CH4is directly proportional to the intensity of ventilation process of the subsurface atmosphere. The coloured points correspond to paired data on the average concentrations of both parameters in the underground air for each field campaign of spot air sampling. Three main caves were considered to display this functional relationship, namely, Castañar, Altamira and Ojo Guareña. Continuous monitoring of radon activity in the underground air was conducted in these caves. Thexaxis for radon concentration in underground air is divided into two parts (with linear and logarithmic scale, respectively) to show the variations of the ratio of the concentrations of CO2and CH4in a very broad range of radon activity. The continuous black line corresponds to a second-order hyperbola that best fits the functional relationship between the ratio of the concentrations of both the greenhouse gases (CO2and CH4, in p.p.m.) and its radon activity (222Rn in Bq m−3), ([CH4]·[CO2]−1)·1,000=4.108 × 105·([222Rn] +0.045)−1, withR2=0.96). Figure 6: Variation in the ratio of the concentrations of both greenhouse gases in underground air in relation to radon activity. The ratio of the concentrations of CO 2 and CH 4 is directly proportional to the intensity of ventilation process of the subsurface atmosphere. The coloured points correspond to paired data on the average concentrations of both parameters in the underground air for each field campaign of spot air sampling. Three main caves were considered to display this functional relationship, namely, Castañar, Altamira and Ojo Guareña. Continuous monitoring of radon activity in the underground air was conducted in these caves. The x axis for radon concentration in underground air is divided into two parts (with linear and logarithmic scale, respectively) to show the variations of the ratio of the concentrations of CO 2 and CH 4 in a very broad range of radon activity. The continuous black line corresponds to a second-order hyperbola that best fits the functional relationship between the ratio of the concentrations of both the greenhouse gases (CO 2 and CH 4 , in p.p.m.) and its radon activity ( 222 Rn in Bq m −3 ), ([CH 4 ]·[CO 2 ] −1 )·1,000=4.108 × 10 5 ·([ 222 Rn] +0.045) −1 , with R 2 =0.96). Full size image It is widely known that the photochemical oxidation of CH 4 in the troposphere is largely dominated by its reaction with hydroxyl radicals (OH). Under the majority of environmental conditions, the hydroxyl radical lifetime is less than a second [44] . Unlike the outdoor atmosphere, however, one of the important OH sources in indoor air may be from radioactive 222 Rn decay. An earlier study provided basic data for the evaluation of indoor radioactive pollution using chemical amplification techniques [45] , quantifying the HOx production rate in indoor air from the radiolysis of water vapour by radon decay on an average rate of (4.31±0.07) × 10 5 HOx molecules per radon decay per second (Bq) over a range of relative humidity from 3.4 to 55.0% at 22 °C. The ionic reactions of gaseous CH 4 with its each primary ion, including ions CH 4 + , CH 3 + , CH 2 + , CH + and C + , represent other mechanism of CH 4 removal. An ion-molecule reaction mechanism is implicated in the formation of these upper homologues of CH 4 , according to [46] , [47] : The starting point of this ion-molecule reaction mechanism is the CH 4 + ion, which also appears under the action of uranium–radon (and its descendants) α-attack of CH 4 (ref. 48 ). In the case of ion-molecule reactions of O + with CH 4 , other product ions are generated, such as OH − and CH 4 + (ref. 49 ). Therefore, the above-mentioned reactions for CH 4 removal by oxidation with hydroxyl radicals and ion-molecule reactions provide feedback to the system. Overall, our findings contribute to a conceptual advance in our understanding of the CH 4 budget by including the subsurface-related CH 4 sink, which has long been largely overlooked. The discovery of frequent (daily), rapid (several hours) and complete CH 4 consumption in subsurface locations makes the uppermost portion of the vadose zone a special site for a CH 4 sink. CH 4 concentrations in underground air below the atmospheric background were found at all points inside the group of caves that was studied. In addition, rapid consumption of atmospheric CH 4 was observed in the underground air of dynamically ventilated caves (for example, Altamira Cave), just after the advective mixing of the cave air with exterior air. Therefore, sub-atmospheric CH 4 concentrations have not only been observed locally but are widespread the atmospheres of all the studied caves. The caves that were studied are distributed across a range of latitudes from 36–43° N to 0–5° W ( Supplementary Fig. 1 ; Supplementary Table 1 ) and they have different geomorphological properties, different locations relative to the surface and different host-rock discontinuities. Our in situ measurements have also documented the link between CH 4 depletion and ion concentration in the subsurface atmosphere; however, the mechanism of CH 4 consumption remains a hypothesis to be tested by laboratory experimentation. In light of these results, a new line of research could extrapolate to a global scale and analyse the CH 4 sink that has been described here for the subterranean atmosphere. There are early observations regarding CH 4 sinks in cave atmospheres that refer to other latitudes in the southern hemisphere, which are quite different to the locations in the north temperate zone that are described here. The phenomenon described here may thus be relevant on a global scale. CH 4 consumption of 1,000 p.p.b. in only a few hours was described in the subterranean air of an Australian cave, for example [26] . There are not yet enough globally representative data on CH 4 in subsurface atmospheres, so extrapolation of the CH 4 -sink model to a global scale still entails much uncertainty. Part of what is estimated at present to be soil uptake may be due to subsurface atmosphere; therefore, the CH 4 sink suggested here is probably at present embedded in the soil uptake term of forward and inverse modelling studies. However, understanding the processes that control the generation, abundance and fate of CH 4 in the atmosphere, oceans and shallow crust is critical for understanding the future of the environment, because CH 4 is a naturally and anthropogenically emitted GHG [50] . Improved knowledge about the oxidation of CH 4 in the subsurface atmosphere under temperature and pressure conditions characteristic of the troposphere near sea level (+15 °C and 103.15 kPa, respectively), could lead to the development, in the medium and long term, of technological alternatives for the removal or storage of GHGs, the identification of new cost-effective ways and methods for mitigation CH 4 emissions and the design of new strategies for atmospheric CH 4 elimination in underground environments. Therefore, different formation, transport and removal processes of CH 4 often impart distinctive isotopic fractionations and abundance of clumped isotopologues [51] , which can provide information about the mechanisms involved and determine constraints on the sinks that can help guide future mitigation efforts. Finally, laboratory experiments should be conducted to attempt to reproduce the oxidation of CH 4 under different environmental conditions. Environmental monitoring networks at fieldwork sites Previous studies have demonstrated the availability of a wide set of facilities and devices that are especially designed to control, measure and analyse interesting parameters related to variations in cave environment conditions at each fieldwork site [16] , [17] . Further descriptions, technical data and results from the monitoring networks are found in these reports. These monitoring networks include sensors and data loggers continuously record local environmental parameters in cave air (pressure, temperature and relative humidity, wind speed and direction, air pressure and CO 2 and 222 Rn contents), soil (CO 2 , temperature and moisture content) and the exterior atmosphere (rainfall, temperature, relative humidity, atmospheric pressure, solar radiation, wind speed and direction). GHGs monitoring A specific sampling and analysis programme for GHGs was implemented for each field site, including: (1) seasonal spot air-sampling and GHG analyses during short surveys at all fieldwork sites and (2) intensive field campaigns conducted for 38 h in the Castañar and Altamira caves, to obtain daily cycles of the GHG mixing ratio through comprehensive real-time logging using CRDS. Spot air sampling was conducted seasonally in a predefined network of points spatially distributed inside each cave and during several short surveys (<3 h long). In total, 1,037 air samples were analysed for the seven caves studied, including 549 samples from cave air, 281 samples from soil air and 207 samples from atmosphere. Sampling was duplicated (morning/afternoon) in the most accessible and smaller caves. Exterior and soil air were sampled at fixed locations throughout the day, and, preferably, during maximum (midday) and minimum photosynthetic activity (early morning). Cave and atmosphere samples were taken 1 m above from the floor. Soil air collection was conducted at sites located vertically above each cave using a steel tube with grooved sides at its ends. The tubes were inserted to a depth of 20–50 cm near the bedrock–soil interface. Soil air was extracted using a micro-diaphragm gas pump (KNF Neuberger, Freiburg, Germany) at 3.1 l min −1 at atmospheric pressure, and the pump was equipped with a 0.2-μm filter to avoid contamination with airborne particles. A portable air compressor (AQUANIC s790) was run at 0.4 l min −1 for the cave air and atmosphere samples. Air samples were collected into 1L Tedlar bags with lock valves, especially designed to ensure the inertness and impermeability of air samples. Each air sample was purged at least one time with air from each sampling point to avoid contamination. Furthermore, the operator remained at a sufficient distance from the portable air compressor during the short interval needed for filling each 1L Tedlar bag, thereby avoiding any contamination by human breathing. The Picarro analyser works with a sample flow rate below 0.05 s.l.m. (standard litre per minute, at 760 Torr) and it is only necessary 10 min for achieving a reliable measurement of the three parameters (CO 2 , CH 4 and δ 13 CO 2 ), therefore <50 s of pumping is enough to provide a suitable volume of air (both from cave and exterior atmospheres) for subsequent analysis using the CRDS technique. Less than 20 s of pumping was enough to provide a suitable volume of soil air for subsequent analysis using the CRDS technique. Thus, we ensured that no air was taken in from the atmosphere. The bag samples were analysed within 48 h of sampling to determine CO 2 and CH 4 concentrations and the isotopic δ 13 CO 2 signal using a laser-based analyser that employs CRDS technology [52] , as described below. In situ and real-time measurements of CO 2 , CH 4 and δ 13 CO 2 were carried out during an intensive field campaign of 38 h using a field-deployable CRDS analyser model G2101-i (Picarro Inc., Santa Clara, CA, USA). This fieldwork aimed to provide detailed records of GHG variations on short-term and diurnal timescales. Continuous monitoring of GHGs was conducted in the Altamira cave, for which a previous complete environmental database regarding cave processes exists. The field campaign was deployed during the warm, dry period at the end of the summer, when the cave is most tightly coupled with the external atmosphere and ventilation is at its most effective [24] , [25] . A detailed time series of GHGs content was obtained (>1,18,000 records with data of 12 CO 2 and 13 CO 2 contents every 2 s), covering a monitoring period of 38 h (two night-time periods and one daytime period, from day 19 until 21 September 2011). The δ 13 C–CO 2 value was automatically calculated using the CRDS analyser by the raw measurements of 12 CO 2 and 13 CO 2 concentration and by taking a central moving average with a window of 5 min, which provides suitable precision according to the manufacturer’s specifications. In addition, a comprehensive network of monitoring stations was specifically implemented to register the coeval short-term environmental changes, including parameters such as air temperature, relative humidity, air pressure and radon contents. The CRDS analyser was operated in continuous mode with a network of tubes connected to a multivalve sequencer, which enabled simultaneous air sampling from different locations (cave, soil and atmosphere) for >10 min each time by alternating the opening and closing of valves. Air from each location was pumped using a 4-mm (inner diameter) polyurethane tube from the main galleries of each cave site and using a micro-diaphragm gas pump as described above. An air extraction tube was connected to the analyser using a T-connection to avoid problems related to overpressure effects. As an alternative to continuous gas monitoring, sampling bags of exterior and soil air were also collected throughout the day. Analyses of GHGs using both the procedures (spot-sampling bags and continuous real-time monitoring) were performed using a CRDS analyser Picarro G2101-i (Picarro Inc.). This analyser performs in situ and real-time measurements of atmospheric levels of carbon dioxide ( 12 CO 2 and 13 CO 2 ), CH 4 and water vapour (H 2 O v ). The isotopic δ 13 CO 2 relationship is automatically measured as a calculation based on 12 CO 2 and 13 CO 2 concentrations and considering a correction due the presence of other target species (CH 4 and H 2 0 v ). Precisions of 200 and 10 p.p.b. are guaranteed by the manufacturer for 12 CO 2 and 13 CO 2 , respectively, over a wide operating range, with a resulting precision of <0.3‰ for δ 13 C(CO 2 ) after 5 min of analysis. The maximum drift of δ 13 C(CO 2 ) is <2.0‰ over 24 h at standard air pressure (peak to peak, 1 h average). Periodic tests were conducted to check that the analyser achieved the above performance specifications (precision and drift) in accordance with the guidelines of the manufacturer (test for 24 uninterrupted hours using the analyser attached to a cylinder of compressed air with known GHG abundances). Measurements of CO 2 in air were performed relative to three reference standards whose gas mixing ratio was determined with high precision and accuracy. On each day/session of analysis using the CRDS analyser (field deployment or analysis of air bags in the lab), the internal secondary standards were run regularly, at least at the beginning and at the end of the analyses, to verify the proper functioning of the analyser. This procedure periodically confirmed that the performance specifications regarding CO 2 analyses via CRDS were met. Regarding CH 4 measurements, the instrument’s response to the sample was also compared with three standards with known CH 4 contents. The measurement accuracy determined through repeated analysis of CH 4 in standard gas cylinders was <0.1 p.p.m. in the studied range of levels (0–2 p.p.m.). In addition, CH 4 measurements was corrected as a function of the presence of H 2 0 v through periodical calibrations of the analyser using synthetic gases with known CH 4 abundances (0, 0.5 and 1.7 p.p.m.v.) over a wide range of H 2 0 v levels (0–3.5%). In addition, some initial spot measurements of air ion density were conducted in Castañar cave to test the range of values in underground air with null CH 4 concentration. A handled air ion counter was used (AlphaLab Air Ion Counter). This instrument is a true ion density metre, based on a Gerdien Tube (Gerdien Condenser) design, and it contains a fan that pulls air through the metre at a calibrated rate. The Air Ion Counter is designed to measure density of ions, that is, the number of ions per cubic centimetre in air, accomplishing the following performance specifications: range: 0–2 × 10 7 ions per m 3 ; resolution: 10 ions per m 3 ; accuracy:±25% of the reading; and response time: 2 s. It also measures this number separately for positive and negative ions. In light of these preliminary observations, a detailed multiparametric and spatially resolved monitoring of air ions density was conducted during a specific field survey in Ojo Guareña cave, in tandem with the analysis of gas composition (CH 4 , CO 2 and δ 13 C–CO 2 ) and microclimatic parameters (temperature and relative humidity) in the underground air, the soil air and the external atmosphere. For this study, continuous monitoring (every half hour) of changes in the radon concentration in the underground air was conducted at three cave sites: Castañar, Altamira and Ojo Guareña. Several Radim 5WP monitors (SMM Company, Prague, Czech Republic and distributed by GT-Analytic KG Innsbruck, Austria) were used, because these monitors are mainly designed for indoor radon measurements. These monitors determine radon concentration by measuring gross α-activity of the radon decay products 218 Po and 214 Po, which are collected electrostatically on the surface of a Si-semiconductor. The lowest activity detectable is 80 Bq m − 3 for 1-h measurements with a statistical error equal to ±20%. The maximum detectable activity is 150 kBq m − 3 . The instrument response is 0.4 (imp h −1 )/(Bq m − 3 ). The monitors were periodically calibrated by the manufacturer. In addition, the monitors were checked regularly in the field (inside the caves) using a Pylon AB5 scintillator photomultiplier with a continuous passive radon detector (Pylon Electronics Inc., Ottawa, Canada) as a reference instrument. This reference instrument was periodically calibrated to provide highly accurate measurements (lowest detectable activity: 24.8 Bq m −3 , with a sensitivity of 0.041 c.p.m. (Bq m −3 ) −1 , accuracy of ±4% and nominal background of 0.4 c.p.m.). MOBs tracking Microbiological sampling was conducted to assess the presence or absence of MOBs in the edaphic profile at exterior and sediments and rock surfaces into cave from each monitored field site. Inside caves, samples were collected in the cave entrance and in the most remote but accessible locations. Sampling was carried out using sterilized materials. On collection, the samples were stored on ice and processed on arrival to the laboratory. Collected samples were analysed by an ordered set of techniques: nucleic acid extraction and PCR amplification, cloning and sequencing and sequence analyses [53] . Nucleic acid extraction and PCR amplification . Extraction of total nucleic acids from the samples was performed using the method proposed by Griffiths et al. [54] in conjunction with a FastPrep instrument, according to the manufacturer’s instructions. Extracted nucleic acids were resuspended in 50 ml of sterile ultrapure water (Sigma-Aldrich). For RNA extraction, a 25-ml aliquot was subjected to a DNase digestion step using a RNase-Free DNase (Qiagen), and the purification of RNA using the RNeasy MinElute Cleanup kit (Qiagen), according to the manufacturer’s instructions. Superscript II Reverse Transcriptase (Invitrogen) was used to synthesize complementary DNA (cDNA) using specific primers: Mb661 (5′-CCG GMG CAA CGT CYT TAC C-3′) and A682 (5′-GAA SGC NGA GAA GAA SGC-3′) for bacterial pmoA gene [55] , [56] and 1492R (5′-GGY TAC CTT GTK WCG ACT T-3′) for bacterial 16S rRNA gene [57] at a temperature of 42 °C for 50 min. Amplification of cDNA will be performed with the methanotrophs-specific primer pairs: A189F (5′-GGN GAC TGG GAC TTC TGG-3′)/Mb661, and A189F/A682 (ref 55 ), and a universal bacterial primer: 27F (5′-AGA GTT TGA TCC TGG CTC AG-3′)/1492R (ref 56 ). One or 2 ml of cDNA, diluted 1/10 was used as a template. PCR conditions were the same for DNA. PCR reactions were performed in a Bio-Rad iCycler thermal cycler (Bio-Rad). The PCR reaction mixture (1 ml) contains 100 ml of PCR buffer (Biotools), 30 ml of MgCl2 (50 mM, Biotools), 10 ml of each primer (50 mM), 100 ml of dNTPs (100 mM, Bioline), 5 ml of Taq polymerase (Biotools) and 750 ml of sterile ultrapure water. The thermal cycler for PCR amplification consisted of 94 °C for 4 min; 28 cycles of 94 °C for 1 min, 56 °C for 1 min (45 °C for 27F/1492R), 72 °C for 45 s; and a final step of 72 °C for 5 min. Positive and negative controls were included in all amplification experiments. All amplification products were purified using a JETquick PCR Purification Spin kit (Genomed) and stored at −20 °C for further analysis. Cloning and sequencing DNA libraries of PCR amplified products were constructed using the pGEM-T Easy Vector (Promega) and then transformed into One Shot Max Efficiency DH5a-T1 chemically competent Escherichia coli (Invitrogen) according to the manufacturer’ instructions. Transformants were randomly picked and transferred to other plates containing Luria–Bertani medium supplemented with 100 mg ml −1 ampicillin and 15% w/v glycerol and stored at −80 °C. The amplicons that contain the correct size of pmoA and 16S rRNA genes fragment were re-amplified using the primer pairs as described above. On average, 100 clones from each library were sequenced at Macrogen Inc., Korea. Sequence analyses Low-quality (short) sequences were removed from the data set. Sequences were aligned using the software package _other [58] . Sequences were checked for chimera by chimera.slayer as implemented in _other . Putative chimeric sequences were excluded from further analysis. After this analysis, all sequences were compared with the non-redundant database of sequences deposited at the National Center for Biotechnology and EzTaxon [59] using BLASTN algorithm [60] . Aligned sequences were clustered into operational taxonomic units using _other , with a 97% sequence identity cutoff for 16S rDNA sequence and 93% for pmoA sequence [61] . Rarefaction curves and Venn diagrams were also obtained using _other. How to cite this article: Fernandez-Cortes, A. et al. Subterranean atmospheres may act as daily methane sinks. Nat. Commun. 6:7003 doi: 10.1038/ncomms8003 (2015).